Multiple enzymatic activities of ParB/Srx superfamily mediate sexual conflict among conjugative plasmids Conjugative plasmids are typically locked in intergenomic and sexual conflicts with co-resident rivals, whose translocation they block using fertility inhibition factors (FINs). We describe here the first crystal structure of an enigmatic FIN Osa deployed by the proteobacterial plasmid pSa. Osa contains a catalytically active version of the ParB/Sulfiredoxin fold with both ATPase and DNase activity, the latter being regulated by an ATP-dependent switch. Using the Agrobacterium tumefaciens VirB/D4 type IV secretion system (T4SS), a relative of the conjugative T4SS, we demonstrate that catalytically active Osa blocks T-DNA transfer into plants. With a partially reconstituted T4SS in vitro , we show that Osa degrades T-DNA in the T-DNA-VirD2 complex before its translocation. Further, we present evidence for conservation and interplay between ATPase and DNase activities throughout the ParB/Sulfiredoxin fold, using other members of the family, namely P1 ParB and RK2 KorB, which have general functional implications across diverse biological contexts. DNA transfer systems, such as the subfamily of the type IV secretion systems (T4SSs) designated as the conjugation machines, play a major role in horizontal gene transfer and spread of fitness-enhancing adaptations in bacterial populations [1] , [2] . During conjugation, a mobile DNA element is processed as a single-stranded transfer intermediate termed the T-strand or T-DNA, which is then delivered through the ‘mating’ channel to a recipient cell. The mating channel spans the donor cell envelope and is assembled from a dozen or more subunits, termed the ‘mating pair formation’ proteins (VirB1-VirB11), and a coupling factor (T4CP), VirD4, that serves to link the DNA substrate with the channel [3] , [4] , [5] , [6] . Majority of mobile genetic elements in Gram-negative bacteria encode conjugation systems composed of a core set of mating pair formation subunits and T4CPs bearing phylogenetic similarities to those of the VirB/VirD4 T4SS of Agrobacterium tumefaciens [7] . A. tumefaciens uses the VirB/VirD4 T4SS to deliver oncogenic T-DNA and protein effectors to plant cells to induce a tumorous growth termed crown gall disease [8] , [9] , [10] . Conjugative plasmids are locked in genomic conflicts with other co-resident plasmids. Consequently, they often encode and deploy fertility inhibition factors (FINs) to selectively block conjugative transfer of ‘rival’ co-resident plasmids [11] , [12] , [13] . Among these poorly understood FINs, Osa, encoded by the IncW plasmid pSa is an oncogenic suppressor that renders the Ti plasmid-containing A. tumefaciens nearly avirulent [14] , [15] . A homologous FIN, FiwA, encoded by plasmid RP1 (IncPα), blocks the transfer of the co-resident plasmid R388 of incompatibility group IncW [11] . Studies to date have suggested that Osa blocks T-DNA and VirE2 transfer from Agrobacterium to the plant cell without affecting T-strand generation or VirB/D4 T4SS assembly [16] , [17] , [18] . However, molecular mechanisms underlying the action of Osa and homologous FINs remain unknown. Hence, to elucidate the mechanism of action of Osa-like FINs, we first solved the crystal structure of Osa. This allowed functional characterization of the active site of Osa, which supports both ATPase and DNase activities. The model for Osa’s action derived from these findings has far-reaching implications for diverse biological systems containing members of the ParB/Srx superfamily. Osa structure and predicted active site Osa crystals of P4 3 2 1 2 space group diffracted up to 1.75 Å. As structures of Osa’s close relatives are unavailable, we solved its structure using the single anomalous dispersion method with KAu(CN) 2 for phasing. 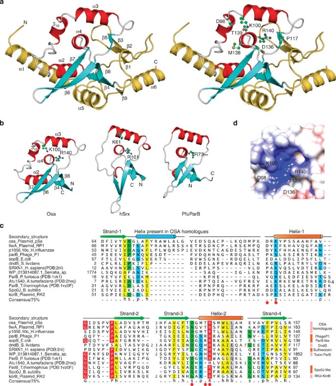Figure 1: Crystal structure of Osa with predicted active site residues. (a) Cartoon representation of Osa (left) showing the position of conserved residues (right). Helices and strands corresponding to the conserved structural core of the ParB/Sulfiredoxin fold are in red and cyan respectively. Additional lineage-specific structural elements are coloured golden yellow. (b) Conserved structural core of the ParB/Sulfiredoxin fold: Osa (64–158), human Sulfiredoxin (hSrx:12–91, PDB:2rii) and ParB (Spo0J) fromP. furiosus(Pfu ParB:16–90, PDB:1vk1). (c) Multiple sequence alignment of the ParB/Srx superfamily. Predicted active site residues are shown as red circles. Sequences are labelled by their gene and species names. The alignment is coloured based on 75% consensus using the following scheme; p: polar residues (CDEHKNQRST) shaded blue, h: hydrophobic (ACFILMVWY) residues shaded yellow, s: small (ACDGNPSTV) residues shaded green and big (QRKEILMWYF) residues shaded grey. Absolutely conserved residues are shaded red. Secondary structure is shown above the alignment with the core ParB/Srx strands in green and helices in orange. The blue helix is only conserved in Osa homologues. (d) Electrostatic surface representation of the predicted active site of Osa is shown with putative active site residues marked. The overall structure of Osa, refined to a final R and R free of 19.7 and 23.9, respectively ( Table 1 ), contains a compact globular domain (~60 × 40 × 36 Å) with six α-helices, one η-helix (3 10 ) and two β-sheets ( Fig. 1a , Supplementary Fig. 1a ). Structural comparison using DALI [19] recovered human Sulfiredoxin (hSrx) and several ParB-like proteins ( Z ~4.5). Further visual examination of the topology confirmed that Osa belongs to the ParB/Srx superfamily. The conserved core ParB/Srx fold, including the version seen in Osa, is a distinctive structure with four strands and two helices ( Fig. 1a,b , Supplementary Fig. 1b ); β4-α2-3 10 helix-α3-β6-β7-α4-β8. Of these, the second conserved helix (α4) contains the arginine residue (R140), which is highly conserved throughout the ParB/Srx fold ( Fig. 1c ), with remaining conserved structural elements forming a ring around that helix ( Fig. 1a ). In addition, the extended linker between the first helix (α2) and the β-hairpin (β6–β7) in the core of the ParB/Srx fold has a small residue (usually proline; P117 in Osa) whose backbone carbonyl group forms a polar contact with the guanidino group of the conserved arginine to position it in a cavity reminiscent of an active site ( Fig. 1a,d ). Table 1 X-ray data collection and refinement statistics. Full size table Figure 1: Crystal structure of Osa with predicted active site residues. ( a ) Cartoon representation of Osa (left) showing the position of conserved residues (right). Helices and strands corresponding to the conserved structural core of the ParB/Sulfiredoxin fold are in red and cyan respectively. Additional lineage-specific structural elements are coloured golden yellow. ( b ) Conserved structural core of the ParB/Sulfiredoxin fold: Osa (64–158), human Sulfiredoxin (hSrx:12–91, PDB:2rii) and ParB (Spo0J) from P. furiosus (Pfu ParB:16–90, PDB:1vk1). ( c ) Multiple sequence alignment of the ParB/Srx superfamily. Predicted active site residues are shown as red circles. Sequences are labelled by their gene and species names. The alignment is coloured based on 75% consensus using the following scheme; p: polar residues (CDEHKNQRST) shaded blue, h: hydrophobic (ACFILMVWY) residues shaded yellow, s: small (ACDGNPSTV) residues shaded green and big (QRKEILMWYF) residues shaded grey. Absolutely conserved residues are shaded red. Secondary structure is shown above the alignment with the core ParB/Srx strands in green and helices in orange. The blue helix is only conserved in Osa homologues. ( d ) Electrostatic surface representation of the predicted active site of Osa is shown with putative active site residues marked. Full size image Using structure-guided sequence alignment ( Fig. 1c , Supplementary Fig. 1c ), we identified four other residues of Osa, K100, D98, D136 and T139 that are highly conserved among other Osa-like FIN factors FiwA, and ICE1056Fin. Importantly, these five conserved residues, R140, K100, D98, D136 and T139, are located in close proximity around the axis of the second conserved helix (α4) of the ParB/Srx fold in a charged pocket that is conserved throughout the superfamily ( Fig. 1d ). Hence, we hypothesized that this cavity is potentially the active site of Osa that is responsible for its FIN activity. In vivo analysis of Osa To demonstrate FIN activity of Osa in vivo , we used the agroinfiltration method [20] to monitor T-DNA transfer through the Agrobacterium VirB/D4 T4SS into plant cells. To test the functional importance of the predicted active site of Osa in vivo , we generated osa - K100A , osa - R140A , osa - K100A-R140A (Osa-KR) and osa-D98A-K100A-D136A-T139A-R140A (Osa-penta) mutants ( Supplementary Tables 1 and 2 ). Native and mutant versions of Osa were co-transformed into Agrobacterium LBA4404 with a plasmid-borne GUS reporter bearing an intron. On agroinfiltration, the GUS reporter-based bioassay [21] showed that the single mutations (K100A; R140A) partially blocked T-DNA transfer through VirB/D4 T4SS ( Fig. 2 ). However, Osa-KR and Osa-penta mutants failed to block T-DNA transfer into Nicotiana cells indicating complete loss of biological activity. As expected, native Osa completely blocked T-DNA transfer. 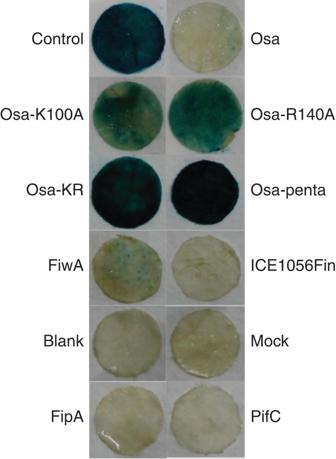Figure 2: Active site of Osa is essential for T-DNA transferin vivo. Results of GUS (β-glucuronidase) assay after agroinfiltration ofNicotiana tabaccumleaf discs are shown. Blue-green colour indicates GUS expression, and thus transfer ofgusgene flanked with T-DNA borders fromAgrobacteriuminto plant. Blank:Agrobacteriumresuspension buffer, Mock:Agrobacterium tumefaciensLBA4404 strain alone, Control: LBA4404 containing pCAMBIA1301 and pSoup vector alone, without any insert. Test experiments hadAgrobacteriumclones harbouring pCAMBIA1301 and pSoup containing either Osa or one of its mutants, or other FINs—ICE1056Fin, FipA and PifC. Figure 2: Active site of Osa is essential for T-DNA transfer in vivo . Results of GUS (β-glucuronidase) assay after agroinfiltration of Nicotiana tabaccum leaf discs are shown. Blue-green colour indicates GUS expression, and thus transfer of gus gene flanked with T-DNA borders from Agrobacterium into plant. Blank: Agrobacterium resuspension buffer, Mock: Agrobacterium tumefaciens LBA4404 strain alone, Control: LBA4404 containing pCAMBIA1301 and pSoup vector alone, without any insert. Test experiments had Agrobacterium clones harbouring pCAMBIA1301 and pSoup containing either Osa or one of its mutants, or other FINs—ICE1056Fin, FipA and PifC. Full size image We also tested and found that Osa homologues including FiwA from RP1 and FIN p1056.10c (ICE1056Fin) encoded by an integrative and conjugative element of Haemophilus influenzae (ICEHin1056) (ref. 22 ) similarly blocked T-DNA transfer ( Fig. 2 ). Thus our in planta experiments demonstrated that Osa and its two homologues require their cognate ParB/Srx-type active sites to block T-DNA transfer. Osa exhibits ATPase and DNase activities To understand how the predicted active site of Osa might relate to its biological function, we investigated its biochemical activities in vitro . Accordingly, we tested if ParB/Srx fold-mediated biochemical functions are conserved among Osa and other FINs. Pyrococcus furiosus ParB, a member of the superfamily possesses DNase activity [23] , while another member, Arabidopsis thaliana Srx, possesses DNase activity and sulfinic acid-reducing activity, which requires ATP-dependent phosphotransfer [24] . Structural superpositions showed that key residues in the inferred active site pocket of human Srx (hSrx: K61, G97, R101) are conserved in Osa (K100, G137, R140) ( Supplementary Fig. 2a ) and located in the above-identified active site. We hence tested if this catalytic site might support ATPase activity, by using Osa and its mutants and a thin layer chromatography (TLC)-based assay to monitor γ-phosphate release. Native Osa readily hydrolysed ATP, and the predicted active site mutations abolished the ATPase activity ( Fig. 3a ). Likewise, Osa homologues ICE1056Fin, P1 ParB and RK2 KorB also exhibited comparable ATPase activity ( Fig. 3a ). Osa hydrolysed ATP and exhibited no comparable GTPase activity. 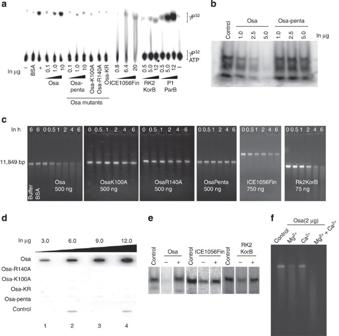Figure 3: The active site of Osa catalyzes both DNase and ATPase activities, and is controlled by an ATP-dependent regulatory switch. (a) ATPase activity: TLC plates were loaded with samples after ATP hydrolysis. Rv3868 ofM. tb, a known ATPase, was used as a positive control. (b) DNase activity: A 90-meric ssDNA was used as a substrate. (c) DNase activity of Osa mutants and various ParB/Srx superfamily proteins using linearized pCAMBIA1301 as the substrate. (d) γ-phosphate retention after ATP hydrolysis: slot blot overlayed with [γ-P32]ATP. The control lanes were loaded with 1: BSA, 2,4: Cdk2/Cyclin E kinase (Abcam). Slots overlayed with [α-P32]ATP did not show comparable bound radioactivity, confirming bound γ-Phosphate. (e) The ATP-dependent switch in Osa, ICE1056Fin and RK2 KorB: nuclease reactions were performed using labelled 90-mer ssDNA substrate with 5–10 μg of proteins for 6 h at 37 °C and loaded onto 4–16% TBE-PAGE. ‘−’ and ‘+’ indicate the absence and presence of 10 mM ATP in the reaction mix. (f) Metal-ion dependency of Osa DNase activity. Osa shows optimal DNase activity in the presence of magnesium ion than calcium. Figure 3: The active site of Osa catalyzes both DNase and ATPase activities, and is controlled by an ATP-dependent regulatory switch. ( a ) ATPase activity: TLC plates were loaded with samples after ATP hydrolysis. Rv3868 of M. tb , a known ATPase, was used as a positive control. ( b ) DNase activity: A 90-meric ssDNA was used as a substrate. ( c ) DNase activity of Osa mutants and various ParB/Srx superfamily proteins using linearized pCAMBIA1301 as the substrate. ( d ) γ-phosphate retention after ATP hydrolysis: slot blot overlayed with [γ-P 32 ]ATP. The control lanes were loaded with 1: BSA, 2,4: Cdk2/Cyclin E kinase (Abcam). Slots overlayed with [α-P 32 ]ATP did not show comparable bound radioactivity, confirming bound γ-Phosphate. ( e ) The ATP-dependent switch in Osa, ICE1056Fin and RK2 KorB: nuclease reactions were performed using labelled 90-mer ssDNA substrate with 5–10 μg of proteins for 6 h at 37 °C and loaded onto 4–16% TBE-PAGE. ‘−’ and ‘+’ indicate the absence and presence of 10 mM ATP in the reaction mix. ( f ) Metal-ion dependency of Osa DNase activity. Osa shows optimal DNase activity in the presence of magnesium ion than calcium. Full size image We next investigated if Osa possesses DNase activity. Assays with both ssDNA and dsDNA substrates showed that native Osa possesses sequence-nonspecific DNase activity, whereas the penta and single mutants were completely inactive ( Fig. 3b,c ). Similarly, ICE1056Fin, RK2 KorB and P1 ParB exhibited DNase activity ( Fig. 3c ; Supplementary Fig. 2b ). The dual ATPase and DNase activities of Osa required Mg 2+ and EDTA treatment abolished both activities ( Supplementary Fig. 2c,d ). Together, our findings establish that Osa and its homologues possess both ATPase and DNase activities and, furthermore, that the active site of Osa is required for both catalytic activities. ATP-dependent regulatory switch in Osa We found that the γ-P 32 O 4 of [γ-P 32 ]ATP bound to Osa, but not to its mutants ( Fig. 3d ). Interestingly, crystal structures of three members of ParB/Srx fold, Osa, Pfu ParB and hSrx have a bound phosphate in their conserved active site pockets ( Supplementary Fig. 2e ). The backbone nitrogens and side chains of T139, R140 in Osa form direct polar interactions with the bound phosphate, whereas the backbone nitrogens of G137, M138 and side chain nitrogen of K100 interact with it via water molecules. Mutation of a phosphate-binding residue from this pocket in hSrx (H100N) resulted in complete loss of activity [25] , [26] . Examination of bound phosphates in these proteins, along with data from our current study, suggests that the γ-phosphate released on hydrolysis can occupy the position occupied by the β-phosphate when ATP is bound to the active site. Given that the γ-phosphate is retained in the active site on ATP hydrolysis across distant members of the ParB/Srx fold, we postulated that phosphate binding plays an important biochemical function. As the ATPase and DNase activities depend on the same active site residues in Osa, we reasoned that availability of ATP could affect its DNase activity, with the retained phosphate potentially blocking DNA binding. To test this, we incubated Osa with its ssDNA substrate with and without ATP in the reaction mixture. While in the absence of ATP Osa showed notable DNase activity, presence of ATP inhibited its DNase activity towards the same substrate ( Fig. 3e ). Similar ATP-dependent inhibition was observed for the DNase activity of ICE1056Fin and RK2 KorB ( Fig. 3e ). On the contrary, presence of plasmid DNA did not affect the ATPase activity of Osa ( Supplementary Fig. 2f ). We also found magnesium to be more conducive for DNase activity than calcium ( Fig. 3f ). These findings suggest that ATP acts as a negative regulatory switch for metal-ion-dependent DNase activity across diverse members of the ParB/Srx superfamily. Osa undergoes multimerization Though Osa was crystallized with one molecule per asymmetric unit, we found it to be in equilibrium with multimeric states in solution even in the absence of substrate DNA ( Supplementary Fig. 3a,b ). When Osa and ICE1056Fin were incubated at 4 °C with either covalently closed circular or linearized dsDNA or ssDNA, they formed nucleoprotein complexes ( Supplementary Fig. 3c ). Increasing concentrations of Osa and ICE1056Fin resulted in increased supershifting of DNA, suggesting that Osa and its homologue ICE1056Fin form higher-order oligomers on binding DNA. It is also apparent from the existing data that ParB and Sulfiredoxin also undergo oligomerization. ParB forms a high-order nucleoprotein complex as it binds repetitive parS sites during pairing of plasmids before partitioning [27] , [28] , [29] . Similarly, Arabidopsis Srx too causes a DNA-mobility shift [24] . These observations suggest that oligomerization upon DNA binding might be a widespread characteristic of members of the ParB/Srx fold. Osa cleaves T-DNA at the VirB/D4 T4SS machine Having characterized its biochemical activities, we tried to place these activities in the larger context of Osa function. Earlier studies showed that Osa fractionates with the membrane [30] and co-localizes in vivo with VirD4, the coupling protein of the A. tumefaciens VirB/VirD4 T4SS [16] . To investigate possible interactions of Osa with relaxosome and/or VirB/D4 T4SS components, we expressed FLAG-Osa in WT A. tumefaciens strain A348 (ref. 31 ), and co-immunoprecipitated its interacting partners using anti-FLAG antibodies. In addition to immunoprecipitating Osa, FLAG-specific antibodies pulled down VirB4 ( Fig. 4a ) and VirB11 ( Fig. 4b ). Such an interaction was neither dependent on the VirD4 coupling protein nor on the assembly of the T4SS machine ( Fig. 4a,b ). Reciprocally, antibodies to VirB4 and VirB11 specifically pulled down FLAG-Osa. To evaluate the in vitro interactions of Osa with T4SS machine and relaxosome components, we first cloned, overexpressed and purified from E. coli soluble forms of the three T4SS ATPases viz VirB4 (425–743 aa), VirB11 (full length) and VirD4 (87–543 aa), and two of the relaxosome components viz VirC1 and VirC2. Next, we tested and confirmed, using TLC assays, that our purified VirB4, VirB11, VirC1 and VirD4 exhibit significant ATPase activities ( Supplementary Fig. 4 ). Again, far-western analyses showed Osa to interact with VirB4 (425–743 aa) and VirB11 ( Fig. 4c ). These results are in clear agreement with the observed in vivo interactions ( Fig. 4a,b ). However, in these conditions, Osa did not interact with VirC1, VirC2 and VirD4. Interestingly, we observed a similar pattern of interaction with ICE1056Fin ( Fig. 4c ). Interaction of both Osa and ICE1056Fin with their cognate T4SS machine components, VirB4 and VirB11 supports a role for this association in plasmid fertility inhibition. 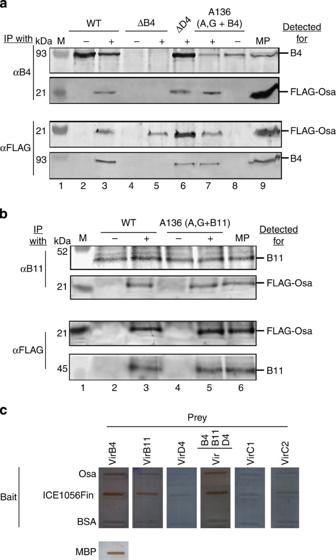Figure 4: Interaction of Osa with VirB/D4 T4SS machine componentsin vivoandin vitro. Forin vivostudy:N,N-Dimethyldodecylamine N-oxide (DDAO)-solubilized membrane protein material immunoprecipitated with (IP with) antibodies to VirB4 ATPase (a) or VirB11 ATPase (b) proteins and FLAG-tag (a,b) listed on the left were analysed for (detected for) proteins listed on the right. Total DDAO-solubilized membrane preparation (MP, right) from the WT (A348) or WT-expressing FLAG-Osa show the position of VirB4/VirB11 and FLAG-Osa, respectively. Absence or presence of FLAG-Osa-expressing plasmid (pKA197) in all strains is indicated by—and+, respectively. Molecular weight markers (M; lane 1) and their sizes in kDa are shown in left. (a) Osa interacts with VirB4 independently of T4S machine and VirD4: Co-immunoprecipitation of VirB4 ATPase and FLAG-Osa in the absence of VirD4 coupling protein and T4S machine. Strains: WT with (lane 3) and without (lane 2) expressing FLAG-Osa (pKA197); ΔB4(PC1004 (virB4knockout (KO)) with (lane 5) and without (lane 4) expressing FLAG-Osa (pKA197); ΔD4(Mx355 (virD4KO) expressing (lane 6) FLAG-Osa (pKA197); A136 (A, G+B4) (KA2002 (WT deleted of pTiA6 plasmid and supplemented with VirA sensory kinase and VirG response regulator) expressing VirB4 (pKA93) with (lane 7) and without (lane 8) producing FLAG-Osa (pKA197). (b) Osa interacts with VirB11 independently of T4S machine and VirD4: co-immunoprecipitation of VirB11 ATPase and FLAG-Osa in the absence of T4S machine. Strains: WT with (lane 3) and without (lane 2) expressing FLAG-Osa (pKA197); A136 (A, G+B11) (KA2002 (WT deleted of pTiA6 plasmid and supplemented with VirA sensory kinase and VirG response regulator)) expressing VirB11 (pSR40) with (lane 5) and without (lane 4) producing FLAG-Osa (pKA197). Forin vitrostudy: (c) Far-western blot of purified MBP fused VirB/D4 T4SS and relaxosome components with purified Osa and ICE1056Fin, probed using horseradish peroxidase-conjugated anti-MBP antibody. Osa and two other FIN factors were used as baits to trap the interacting partner from the T4SS machine and relaxosome. Figure 4: Interaction of Osa with VirB/D4 T4SS machine components in vivo and in vitro . For in vivo study: N , N -Dimethyldodecylamine N-oxide (DDAO)-solubilized membrane protein material immunoprecipitated with (IP with) antibodies to VirB4 ATPase ( a ) or VirB11 ATPase ( b ) proteins and FLAG-tag ( a , b ) listed on the left were analysed for (detected for) proteins listed on the right. Total DDAO-solubilized membrane preparation (MP, right) from the WT (A348) or WT-expressing FLAG-Osa show the position of VirB4/VirB11 and FLAG-Osa, respectively. Absence or presence of FLAG-Osa-expressing plasmid (pKA197) in all strains is indicated by—and+, respectively. Molecular weight markers (M; lane 1) and their sizes in kDa are shown in left. ( a ) Osa interacts with VirB4 independently of T4S machine and VirD4: Co-immunoprecipitation of VirB4 ATPase and FLAG-Osa in the absence of VirD4 coupling protein and T4S machine. Strains: WT with (lane 3) and without (lane 2) expressing FLAG-Osa (pKA197); Δ B4 (PC1004 ( virB4 knockout (KO)) with (lane 5) and without (lane 4) expressing FLAG-Osa (pKA197); Δ D4 (Mx355 ( virD4 KO) expressing (lane 6) FLAG-Osa (pKA197); A136 (A, G+B4) (KA2002 (WT deleted of pTiA6 plasmid and supplemented with VirA sensory kinase and VirG response regulator) expressing VirB4 (pKA93) with (lane 7) and without (lane 8) producing FLAG-Osa (pKA197). ( b ) Osa interacts with VirB11 independently of T4S machine and VirD4: co-immunoprecipitation of VirB11 ATPase and FLAG-Osa in the absence of T4S machine. Strains: WT with (lane 3) and without (lane 2) expressing FLAG-Osa (pKA197); A136 (A, G+B11) (KA2002 (WT deleted of pTiA6 plasmid and supplemented with VirA sensory kinase and VirG response regulator)) expressing VirB11 (pSR40) with (lane 5) and without (lane 4) producing FLAG-Osa (pKA197). For in vitro study: ( c ) Far-western blot of purified MBP fused VirB/D4 T4SS and relaxosome components with purified Osa and ICE1056Fin, probed using horseradish peroxidase-conjugated anti-MBP antibody. Osa and two other FIN factors were used as baits to trap the interacting partner from the T4SS machine and relaxosome. Full size image To explore the action of Osa in a complex with the T4SS components, we reconstituted the fertility inhibition complex in vitro , using a partial T4SS complex consisting of VirB4 (425–743 aa), VirB11 (full length) and Osa or Osa-penta mutant. In the presence of reconstituted partial T4SS machine, Osa degraded T-DNA covalently linked to VirD2 (ref. 32 ), whereas the penta mutant failed to do so ( Fig. 5a–c ). These data suggest that Osa degrades VirD2-linked T-DNA ( Fig. 5d ) even in presence of the T4SS in vitro despite being protected from other nucleases [33] . 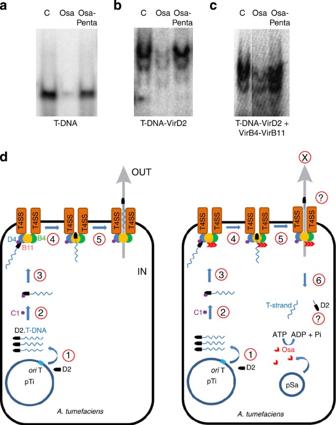Figure 5:In vitroreconstitution of plasmid fertility inhibition and the FIN model. Osa digests naked T-DNA (a), T-DNA linked to VirD2 in the absence (b) and presence of T4SS ATPases VirB4 and VirB11 (c). (d) Proposed model of plasmid fertility inhibition by Osa-like FIN factors. The model on the left illustrates T-DNA transfer during normal conjugation/agroinfection process. In an assumed series of steps, first VirD2 relaxase makes a nick at the 5′ end of right border (RB) sequence, and gets covalently linked to the single-stranded T-DNA (step 1). The T-complex containing T-DNA.VirD2-VirC1 (step 2) docks to the coupling factor VirD4 at the T4SS, through the physical interaction between VirC1 and VirD4 (step 3). Then, the T-DNA docked at the cytoplasmic side of T4SS is channelled through the pore (step 4 and 5). Thereby, the T-DNA substrate is either released in the vicinity or secreted into the cytoplasm of the recipient bacterial host or the plant cell. The model on the right side depicts the possible fate of T-DNA in the presence of an Osa-like FIN factor encoded from a co-resident plasmid pSa. Osa, which is already localized in the vicinity of the membrane, binds to preassembled T4SS through its interaction with VirB11 and VirB4. At this stage, Osa blocks T-DNA transfer through T4SS by two ways (step 4 and step 5): (i) Osa decouples T-DNA from VirD2 through its DNase activity, and (ii) also modulates VirB4-B11-D4 interaction, wherein VirD4 coupling factor loses its affinity to the substrates (step 6). Without VirD2, and also no longer being recognized by VirD4, the decoupled T-DNA cannot hitchhike its way to the other side of the cell. For the sake of clarity, only limited components of T4SS are shown. Figure 5: In vitro reconstitution of plasmid fertility inhibition and the FIN model. Osa digests naked T-DNA ( a ), T-DNA linked to VirD2 in the absence ( b ) and presence of T4SS ATPases VirB4 and VirB11 ( c ). ( d ) Proposed model of plasmid fertility inhibition by Osa-like FIN factors. The model on the left illustrates T-DNA transfer during normal conjugation/agroinfection process. In an assumed series of steps, first VirD2 relaxase makes a nick at the 5′ end of right border (RB) sequence, and gets covalently linked to the single-stranded T-DNA (step 1). The T-complex containing T-DNA.VirD2-VirC1 (step 2) docks to the coupling factor VirD4 at the T4SS, through the physical interaction between VirC1 and VirD4 (step 3). Then, the T-DNA docked at the cytoplasmic side of T4SS is channelled through the pore (step 4 and 5). Thereby, the T-DNA substrate is either released in the vicinity or secreted into the cytoplasm of the recipient bacterial host or the plant cell. The model on the right side depicts the possible fate of T-DNA in the presence of an Osa-like FIN factor encoded from a co-resident plasmid pSa. Osa, which is already localized in the vicinity of the membrane, binds to preassembled T4SS through its interaction with VirB11 and VirB4. At this stage, Osa blocks T-DNA transfer through T4SS by two ways (step 4 and step 5): (i) Osa decouples T-DNA from VirD2 through its DNase activity, and (ii) also modulates VirB4-B11-D4 interaction, wherein VirD4 coupling factor loses its affinity to the substrates (step 6). Without VirD2, and also no longer being recognized by VirD4, the decoupled T-DNA cannot hitchhike its way to the other side of the cell. For the sake of clarity, only limited components of T4SS are shown. Full size image Our findings help elucidate the molecular mechanism of Osa and its homologues in blocking co-resident rival plasmid transmission and A. tumefaciens oncogenicity. Osa degrades T-DNA both when it is crosslinked to the tyrosine of the RCR superfamily relaxase VirD2 ( Fig. 5b ) and when VirD2-bound T-DNA associates with the T4SS inner-membrane complex components in vitro ( Fig. 5c ). These observations together with previous studies suggest that Osa probably acts before T-DNA docking at VirD4 and that it may not target T-DNA until it reaches the T4SS machine [34] , [35] . Overall, our in vitro FIN reconstitution experiments support a model wherein the FINs first localize to the membrane and interact with T4SS machine components encoded by their rival plasmids before degrading the translocating DNA linked to their relaxases ( Fig. 5d ). Interestingly, Osa has also been shown to block the transfer of virulence effector proteins secreted by the Ti plasmid-encoded T4SS, namely VirE2 and VirF [18] , [36] . Physical association of Osa with the above T4SS components could also play a key role in blocking other macromolecular translocations via this system. This also presents a conundrum as to how FIN factors specifically target ‘non-self’ T4SS encoded by the co-resident plasmids as opposed to ‘self’ versions encoded by their own DNA. Indeed a network of non-self plasmid-blocking interactions has been observed for other FINs: FiwA of RP1 (IncPα) blocks pSa (IncW) and FipA of pKM101 (IncN) and PifC of F (IncF) block RP1 (IncP) transfer [11] , [13] , [37] . Our data suggest that FINs might interact specifically with non-self T4SS components. To investigate if other co-factors might be involved in assisting Osa and related FINs in self versus non-self T4SS recognition, we conducted a computational analysis of their genomic contexts to identify conserved gene neighbourhoods or predicted operons. The presence of such conserved operons is a good indicator of interactions between the encoded proteins [38] , [39] . This analysis revealed that Osa and its homologues tend to be encoded in the vicinity of operons encoding transfer-associated or replication-associated genes. These genomic neighbourhoods also include other loci involved in distinct biological conflict systems, such as toxins ( Supplementary Fig. 5a ). We observed that a common denominator in these genomic neighbourhoods is a gene coding for a predicted β-barrel domain typified by the KfrB protein from RK2 plasmid [40] ( Supplementary Fig. 5b ). This domain is either encoded by a gene neighbouring Osa and its homologues (labelled Nuc in the pSa plasmid) or is fused to diverse toxin domains such as DOC (a protein nucleotidyltransferase) [41] , Zeta-toxin (a kinase acting on substrates such as peptidoglycan) [42] and HEPN (a predicted RNase) [43] , [44] . Given these associations ( Supplementary Fig. 5a ), it is conceivable that the KfrB domain plays a key role in discrimination of self from non-self and plays an auxiliary role in aiding Osa to target non-self T4SS. All FINs tested in this study, both those related to Osa, such as FiwA, and ICE1056Fin and unrelated ones namely FipA and PifC blocked T-DNA transfer in vivo ( Fig. 2 ). While Osa and its homologues FiwA and ICE1056Fin are expected to exhibit a similar mechanism, FipA and PifC belong to completely unrelated superfamilies of proteins and probably have their own distinct mechanisms. Moreover, plasmids of the IncPα group also deploy as FINs products of the Ter locus (FiwB) [11] , which has also been implicated as a defensive mechanism against bacteriophages [45] and toxic substances such as Tellurium. The products of the Ter locus are predicted to form membrane-associated complexes that might interfere with fertility of rival plasmids [45] . Thus, we expect a rich diversity of mechanisms to convergently target the T4SS or the DNA substrate as part of the fertility inhibition phenomenon. Our study shows that ATPase and DNase activities are common features across the ParB/Srx superfamily, with retention of the γ-phosphate at the active site and inhibition of DNase activity in presence of ATP. This observation suggests that the DNase activity of Osa-like FINs is likely to be kept in check under normal conditions by the ambient presence of ATP. However, when it associates with the T4SS, the active P-loop ATPases in that complex likely consume ATP creating a local depletion. This in turn might allow unmasking of their DNase activity towards rival T-DNA undergoing transfer. Presence of comparable dual activity across members of the ParB/Srx fold suggests that this might have more general implications for their functions. Members of ParB/Srx superfamily are found in biologically diverse contexts: (1) Cellular genomic-, viral- and plasmid-encoded ParBs are involved in partitioning of their corresponding DNA; (2) Sulfiredoxins restore the activity of oxidized peroxiredoxin in an ATP-dependent manner; they transfer the γ-phosphate to cysteine sulfinic acid in the peroxiredoxin active site with its resultant conversion to a SH group [46] ; (3) Certain recently identified members of the polymorphic toxin systems contain carboxyl-terminal (C-terminal) ParB toxin domains that are predicted to function as nucleases [47] ; (4) DndB and related proteins are involved in regulating DNA phosphorothioation and other recently proposed DNA modifications [48] , [49] ; (5) Certain bacteriophage and related ParB/Srx superfamily proteins are associated with facilitating DNA modifications [48] . Of these, the proteins involved in chromosomal segregation across bacteria (for example, Bacillus subtilis Spo0J, Caulobacter ParB and bacteriophage P1 ParB point to two unifying themes: First, they stimulate the activity of a ParA-like ATPase; second, they possess a C-terminal DNA-binding helix-turn-helix domain with which they can recognize specific sequences at the origins of replicons (ParS sequences). However, current studies on chromosome partitioning [50] , [51] , [52] do not take into account either the DNase or the ATPase activities of ParB. Since we were able to detect both these activities in phage P1 ParB and RK2 KorB, we propose that they are essential for chromosome partitioning. As with Osa, we propose that the DNase and DNA-associating activity of the ParB/Srx domain of these proteins (as opposed to the helix-turn-helix domain) is kept under check by ATP. However, when ATP is locally depleted by ParA(Soj)’s ATPase activity, the DNase and DNA-association activity of the ParB/Srx domain is unleashed, perhaps allowing it to associate with the nucleoid DNA and locally cut it. This in turn might affect its interaction with DNA and explain the observed dynamical reassociation with DNA during segregation. Consistent with this, mutation of a conserved arginine (R80A) in Spo0J, which corresponds to an active site residue in Osa (R140), results in loss of function [53] ( Fig. 1c ). Similarly, the dual activities of other members of the family could also regulate their DNase and DNA-association properties to control DNA modification (for example, DndB) or toxin activity of the polymorphic toxins. In summary, we report the crystal structure of plasmid-encoded FIN Osa. The core of Osa adopts the ParB/Srx fold with a unique active site displaying both ATPase and DNase activity, the latter being negatively regulated by an ATP-dependent switch. Osa degrades Ti plasmid-encoded T-DNA in the T-DNA:VirD2 complex before its translocation through VirB/D4 T4SS machine, a mechanism conserved in Osa-like FINs. Our results offer a unified mechanism that generates testable hypotheses for the roles of a hitherto obscure superfamily of proteins implicated in a wide range of biological functions. Cloning, overexpression and mutagenesis Native Osa, Osa mutants—Osa-KR (K100A-R140A), Osa-penta (D98A-K100A-D136A-T139A-R140A)—and genes encoding FIN factors FiwA, p1056.10c (ICE1056Fin), FipA and PifC, were PCR amplified and cloned into pKA165 (containing p virB ::osa) [16] by replacing osa ( Supplementary Table 1 ). HindIII and KpnI cut, error-free inserts were then mobilized into pSoup for agroinfiltration, and to pETM-41 (EMBL-vector collection) or pET-28a for overexpression in E. coli . PCR cloning and site-directed mutagenesis, using pKA165 as template, was carried out with primers listed in Supplementary Table 2 . Agrobacterium tumefaciens ( A . tumefaciens ) octopine-specific pTiA6-encoded virB4 , virB11 , virD4 , virC1 and virC2 were cloned into InfR-Nhis, and then mobilized into pETM-41 for overexpression. virD2 , P1 parB and RK2 korB were PCR amplified from pTiA6, phage P1 lysate and RP4 plasmid DNA, respectively, and cloned into InfR-Nhis for overexpression. FLAG-Osa was PCR amplified with specific primers ( Supplementary Table 2 ) using pUCD3960 (ref. 18 ) as template. The 0.6-kb amplicon was subsequently cloned into the corresponding sites of pPC914KS+ (ref. 54 ) to obtain pKA197 and finally ligated to the broad host range plasmid pSW172 (Tet R ) [55] . Escherichia coli DH5α was used as the host strain for all plasmid constructions. InfR-Nhis is an in-house modified pRSF-Duet1 vector (Novagen) with In-Fusion (Clonetech) cloning cassette containing TEV protease cleavable N-terminal His 6 -tag. Purification and crystal structure determination of Osa Osa with N-terminal His 6 -tag was purified using Ni 2+ affinity and gel-filtration chromatography, and crystallized using hanging and sitting drop methods at a concentration of 6 mg ml −1 (0.284 mM). Best diffraction quality crystals of Osa were obtained in 8% 2-propanol (v/v), 0.5 M Lithium sulfate, 0.1 M Phosphate-citrate buffer (pH 4.2) and 0.2 M Non-detergent sulphobetaine (NDSB-201). X-ray data sets for native and KAu(CN) 2 -soaked Osa crystals were collected at 100 K using home source fitted with Mardtb image plate (mar345) and a RigakuMicromax 007 rotating anode generator (Cu K α λ =1.5418 Å) operated at 40 kV and 20 mA or R-AXIS IV ++ image plate and FR-E SuperBright rotating anode generator at the National Institute of Immunology, New Delhi. Paratone oil (Hampton Research) and glycerol were used as cryo-protectants. Data were processed using HKL-2000 (ref. 56 ). Phases were calculated using single isomorphous replacement with anomalous scattering method in HKL2MAP [57] . Model building was carried out using Buccaneer [58] , [59] and Coot [60] . Phenix [61] was used for refinement. Ramachandran statistics were checked using PROCHECK [62] . Structural comparison was done using DALI [19] . Figures were made using Chimera [63] and PyMol (Schrödinger, LLC). Multiple sequence alignment Sequence profile searches using the PSI-BLAST [64] programme and the HMMsearch programme of the HMMER3 package [65] were used to identify diverse ParB/Srx homologues. The multiple sequence alignment was generated using Kalign2 (ref. 66 ) followed by manual adjustments based on structural alignments generated by the DALI server. Overexpression and purification of all other proteins Overexpression screening was carried out using various E. coli host strains with appropriate antibiotics in prescribed concentrations, and the ones that yielded optimal amount of target proteins are listed in Supplementary Table 1 . Brief expression and purification protocols for individual proteins are given below. Compositions of the buffer used are in the Supplementary Table 3 . All the prepacked chromatographic columns used in this study are from GE biosciences. Ultracentrifugation devices (Millipore) with various molecular weight cutoff were used for protein concentrations. MBP-Osa and its mutants These proteins were expressed in Rosetta2 (DE3) pLysS strain (Novagen) and purified in four steps, first by amylose affinity, followed by Ni 2+ -affinity, Ion-exchange (HiTrap-Q-HP) and gel-filtration chromatographic columns. Cells grown at 37 °C in Luria–Bertani (LB) broth were induced with isopropyl-β- D -thiogalactoside (IPTG) at OD 600 0.8 and incubated further for 4 h. Cells were sonicated and the clarified lysate supernatant in buffer C, containing 500 mM NaCl, was passed through amylose resin (NEB), equilibrated with the same buffer and eluted with 20 mM D -Maltose. Eluted protein was loaded onto HisTrapFF column charged with Nickel sulphate, washed with buffer A and eluted with buffer B. Salt concentration in the eluted fraction was diluted to 10 mM NaCl, and was loaded onto 5 ml Hitrap-Q-HP column and eluted using a 10–1,000 mM NaCl gradient. Pooled and concentrated fractions were further purified using Hiload 16/60 Superdex S-200 column. ICE1056Fin C-terminal His 6 -tagged protein was expressed in E. coli BL21-CodonPlus cells in LB autoinduction (LB-AI) without trace elements and TB autoinduction media with trace elements (Formedium, UK), respectively. Both secondary cultures were grown at 25 °C for 24 h. Cells were lysed in lysis buffer 1, and the lysate supernatant was loaded onto HisTrapFF Ni 2+ affinity column. The column was washed first with buffer A followed by the same buffer containing 50 mM imidazole and eluted with 250 mM Imidazole. Fractions containing pure target proteins were pooled, concentrated and loaded onto Hiload Superdex S-200 16/60 column preequilibrated with buffer D. VirB11 and VirD4 The overexpression constructs were transformed into E. coli Rosetta2 (DE3) pLysS cells. Cells were grown in LB-AI medium without trace elements at 25 °C for 24 h and lysed in lysis buffer 1, and the lysate supernatant was then gently mixed with amylose resin in batch mode, before packing onto a manual gravity-flow column. Three times the bed volume of buffer E containing 0.05% Triton-X-100 was used to wash off non-specifically bound proteins. Buffer E containing 0.5 mM D -Maltose was used for further washing and then eluted with buffer F. Proteins were further purified using Superdex S-200 16/60 column equilibrated with buffer G. VirB4 VirD4 was expressed in E. coli T7 Express lysY/I q (NEB) cells in LB broth. Cells grown at 37 °C till OD 600 0.6 and then induced with 0.5 mM IPTG at 25 °C for 12 h. Cells lysed in lysis buffer 2 were batch bound to amylose resin, washed with buffer H and eluted with 10 mM maltose. It was then dialyzed against 20 mM Tris–HCl pH 7.4 and 50 mM NaCl. VirC1 and VirC2 These proteins were expressed in E. coli T7 Express I q (NEB) cells using LB broth. Cells grown at 37 °C till OD 600 0.6 were induced with 0.5 mM IPTG and further grown for 5 h. Cells were lysed in lysis buffer 1, and the lysate supernatant was batch bound to amylose resin, washed with buffer E and eluted using buffer F. VirC2 was purified to homogeneity by amylose affinity chromatography, whereas VirC1 needed further purification using HisTrapFF affinity column. Column was washed with buffer A followed by wash with buffer A containing 50 mM imidazole and eluted with 100% buffer B. VirD2 VirD2 was expressed in E. coli BL21-CodonPlus(DE3) cells in LB broth. Cells grown at 37 °C till OD 600 1.0 were induced with 0.5 mM of IPTG and grown further for 12 h at 25 °C. Overexpressed full-length VirD2 was found in the inclusion bodies and a standard protocol was followed for refolding and purification [67] . ParBs RK2 KorB was expressed in E. coli Rosetta 2(DE3) pLysS cells in LB broth. Cells were grown at 37 °C until OD 600 1.0 and then induced with 0.5 mM IPTG at 25 °C for 12 h. Cells were lysed in lysis buffer 1 and the lysate supernatant was passed through 5 ml HisTrapFF column. The column was washed with buffer A and eluted with 75 mM Imidazole. Pure fractions of KorB were pooled and dialyzed into buffer I before passing onto HiTrap-Heparin HP column. Protein was eluted using a gradient run using buffer I and J. KorB eluted around ~140 mM NaCl. P1 ParB was expressed in T7 Express lysY/I q in LB broth. Cells were grown at 37 °C until OD 600 0.6 and then induced with 0.5 mM IPTG for 2 h. Cell lysate supernatant in lysis buffer 2 was passed through 10 ml of chelating sepharose column charged with Co 2+ . Column was washed with buffer K and eluted with a gradient using buffer K and L. Pure fractions were pooled and dialyzed against buffer M to remove excess salt and loaded onto a cation-exchange column (5 ml HiTrap-SP-Sepharose) and eluted using buffer N containing 50 to 1,000 mM NaCl gradient. The N-terminal His-tag was cleaved with TEV protease (20:1 protein to protease ratio) at 20 °C for 16 h. Cleaved His6-tag and the uncut fusion proteins were removed by passing through a 5-ml HisTrapFF column. Pure P1 ParB containing fractions were pooled and passed through GPC column (Superdex S-75 10/60) equilibrated with buffer M. P1 ParB purified to homogeneity was further passed through 5 ml HiTrap-Heparin HP column in buffer I, followed by a gradient run using buffer I and J. ATP binding and hydrolysis Purified proteins were blotted onto nitrocellulose membrane using a multi-well slot-blot manifold, blocked with 5% bovine serum albumin (BSA) at 4 °C for 2 h, washed thrice with PBS containing 0.05% Tween-20 (PBS-T) followed by three washes with PBS (without Tween-20), for 5 min each. Twenty μCi of γ-P 32 radio-labelled ATP in 15 ml of PBS containing 10 mM MgCl 2 was added to the blot and incubated for 30 min. This was followed by three PBS-T washes and then three PBS washes, each for 5 min. The blot was dried and exposed for 12 h and developed using phosphor imager (GE). Slots overlayed with [α-P 32 ]ATP did not show comparable bound radioactivity, confirming bound γ-phosphate. For ATPase assay, proteins were incubated with 0.2 μCi [γ-P 32 ]ATP in the reaction buffer containing 10 mM Tris–HCl pH 8.0, 5 mM MgCl 2 , 50 mM KCl, 2 mM DTT and 80 μg ml −1 BSA. The reactions were carried out for 30 min at 37 °C and then 1.1 μl of the mixture was spotted on polyethyleneimine cellulose TLC plate (Sigma). TLC was run with mobile phase containing 0.5 M LiCl and 1 M formic acid. After the run, TLC plate was air dried and developed using phosphor imager, 2 h after exposure. DNase assay The assays were performed in a 20-μl reaction mixture containing 50 ng linearized dsDNA substrate in nuclease buffer: 50 mM Tris-HCl pH 8.0, 50 mM NaCl, 5 mM MgCl 2 and 3 mM β-ME. The assay mixture was incubated at 37 °C for 4 h and run on 1.0% agarose gel. For DNase assay with ssDNA substrate, a 90-mer oligo ( Supplementary Table 2 ) was commercially synthesized and the 3′ end was labelled with [α-P 32 ]dCTP using terminal transferase (NEB) following manufacturer’s protocol. Aliquots corresponding to 30,000 counts of this labelled ssDNA were incubated with respective proteins for 6 h in the nuclease buffer, with and without different divalent cations and EDTA. Sample aliquots were mixed with protein loading buffer and run on a 4 to 16% gradient TBE-polyacrylamide gel electrophoresis (PAGE), after which the gels were exposed and scanned. Agroinfiltration and GUS assay Agrobacterium tumefaciens LBA4404 strain was co-transformed with pCAMBIA1301 and pSoup constructs containing osa , osa mutants , fiwA , ice1056fin , fipA and pifC , under virB promoter, by electroporation. Transformants were selected on YEM-Agar plates supplemented with 50, 50, 5 and 10 μg ml −1 of kanamycin, streptomycin, tetracycline and rifampicin, respectively. Single colonies were cultured in YEM (Yeast extract-Mannitol) medium supplemented with appropriate antibiotics at 28 °C and at 180 r.p.m. until the cell density reached OD 600 1.0. Cells were harvested and resuspended in infiltration buffer containing 10 mM MES pH 5.7 and 10 mM MgCl 2 at an OD 600 of 0.5. Four to six-week-old leaves of Nicotiana tabaccum were gently infiltrated with the homogenous bacterial suspension using 1 ml syringe, without needle, from the abaxial surface. These leaves were plucked 4 to 7 days after infiltration and tested for GUS activity using 5-bromo-4-chloro-3-indolyl glucuronide (X-gluc) as a substrate in a buffer containing 100 mM Sodium phosphate pH 7.0, 0.5 mM Potassium ferrocyanide, 0.5 mM Potassium ferricyanide, 0.05% Triton-X-100 and 1 mg ml −1 X-gluc [21] . Protein–protein interaction in vivo Using immunoaffinity pulldown, we studied protein–protein interactions between Osa and VirB/D4 T4SS components. Various strains of Agrobacterium tumefaciens were used for this purpose. Here WT refers to A348. A348 is aC58 strain harbouring the octopine-type pTiA6NC plasmid. A348 derivatives include Mx355 (Δ virD4 ) and PC1004 (Δ virB4 ). A136 (A & G) is a C58 strain cured of pTiA6NC plasmid harbouring virA of pTiA6NC and virG of pTiBo542 on its circular chromosome [68] . All A. tumefaciens strains were grown in LB supplemented with glutamate and mannitol at 28 °C. Conditions for induction of the A. tumefaciens vir genes have been described previously [69] . When required, vir -induction medium was supplemented with antibiotics (in μg ml −1 ) as follows: gentamicin (100), tetracycline (5) and carbenicillin (100). Initially, we induced and expressed FLAG-Osa (from pKA197) in 500 ml of A. tumefaciens WT strain A348. Cells were then harvested, lysed by french cell-press treatment and membrane extracts isolated. Two mg of total membrane was then solubilized with N , N -Dimethyldodecylamine N-oxide in 50 mM Tris-HCl, pH 7.4 and 1 mM EDTA, at 4 °C for O/N with gentle rocking. After centrifuging the solubilized material at 15,000 g for 15 min, we used the supernatant and evaluated for Osa interacting partners by co-immunoprecipitation with either antibodies to VirB2 to VirB11, VirC1, VirC2, VirE1, VirE2, VirD1, VirD2 and VirD4 proteins or FLAG-tag. Proteins were resolved by SDS-PAGE as previously described. Vir proteins were transferred to nitrocellulose and later developed with goat anti-rabbit secondary antibodies conjugated to alkaline phosphatase ( Supplementary Fig. 6 ). Since we observed only VirB4 and VirB11 proteins interacting with FLAG-Osa ( Fig. 4a,b ), we further analysed if these interactions were more direct. Consequently, we induced and expressed FLAG-Osa in Δ virB4 , Δ virD4 and A136 (A+G) strains. A136 (A+G) also expressed either VirB4 (pKA93) Fig. 4a or VirB11 Fig. 4b (pSR45) (ref. 31 ). Protein–protein interaction in vitro Purified proteins, Osa and ICE1056Fin, were blotted onto nitrocellulose membrane using a slot-blot manifold blocked with 5% BSA at 4 °C for 1 h, washed thrice with PBS containing 0.05% Tween-20 (PBS-T), followed by three washes with PBS for 5 min each. MBP-tagged purified A. tumefaciens T4SS and relaxosome components-VirD4, VirB11, VirB4 and VirC1 were incubated with immobilized proteins. This was followed by three washes with PBS-T and then three washes with PBS. Horseradish peroxidase-conjugated anti-MBP antibodies, reconstituted in 15 ml of PBS containing 10 mM MgCl 2 , was added to the blot and incubated for 30 min, followed by three PBS-T washes and three PBS washes, each for 5 min. Blots were developed with 3,3′-diaminobenzidine tetrahydrochloride ( Supplementary Fig. 6 ). Oligomerization of Osa BN-PAGE [70] , along with gel-filtration chromatography, was used to assess the oligomeric status of Osa. The protein was incubated with loading buffer for 10 min at room temperature and loaded onto 4 to 20% gradient native PAGE. The gel was run at 100 V at 4 °C. Anode and cathode buffers had the following composition: 100 mM Tris pH 8.0, 40% Glycerol, 0.5% Coomassie Brilliant Blue-G250; 100 mM Tris–HCl pH 8.8; and 100 mM Histidine (pH adjusted to 8.0 using Tris base), 0.02% Coomassie Brilliant Blue-G250, respectively. After the gel was run two-thirds of its length, the cathode buffer was replaced with fresh buffer without the dye. Gel was stained with Coomassie Brilliant Blue R-250 and then destained, as done for regular SDS-PAGE. T-DNA-VirD2 complex preparation Fifteen picomoles of 90-mer oligonucleotides (Macrogen) with and without T-DNA left border (LB) and right border (RB) were labelled at the 3′ end using 30μCi [α-P 32 ]dCTP and terminal transferase. The labelling reaction was carried out for 15 min at 37 °C followed by purification through Illustra MicroSpin G-25 Columns (GE). The purified labelled oligos were quantified for labelling efficiency by measuring the counts in scintillation counter. RB containing 3′ labelled oligo (15 pmol) was covalently attached to VirD2 (100 pmol) at the 5′ end by incubating the mixture at 37 °C for 4 h in a reaction buffer containing 20 mM Tris–HCl pH 8.8, 50 mM NaCl and 5 mM MgCl 2 . Products containing 30,000 counts were loaded onto gradient TAE-PAGE (4–16%) gels using 1 × SDS-PAGE loading dye to check the site-specific covalent modification of oligo by VirD2 and then used in FIN reconstitution. FIN reconstitution Covalently linked T-DNA-VirD2 substrate complex was made using the above protocol. Cytoplasmic complex of the T4SS was reconstituted by mixing VirB4 and VirB11 in 1:1:1 molar ratio, by adding 30 fmol of each protein. This mixture was dialyzed into a buffer containing 25 mM Tris pH 8.0, 100 mM NaCl and 2 mM DTT for 2 h. DNase reaction was set up with radiolabeled VirD2.T-DNA complex (30,000 counts; 30 fmol) in nuclease buffer. Osa and Osa-penta were added to this reconstituted complex, to the final concentration of 3.8, 7.6 and 38 μmol. The reaction mixture was incubated for 6 h at 37 °C and the products were run on 4–16% gradient TAE-PAGE, detected using phosphor imager, after exposure for 2 h. We observed that higher amounts of Osa is required to cleave T-DNA linked to VirD2 and also when T4SS ATPases are present, compared with naked DNA. This is likely to be due to stoichiometric interactions influencing nuclease activity of Osa in vitro . Accession codes : PDB coordinates : The atomic coordinates of Osa native and derivative have been deposited in the Protein Data Bank under accession numbers 4O7K and 4OVB, respectively. How to cite this article: Maindola, P. et al. Multiple enzymatic activities of ParB/Srx superfamily mediate sexual conflict among conjugative plasmids. Nat. Commun. 5:5322 doi: 10.1038/ncomms6322 (2014).